Practical photon number detection with electric field-modulated silicon avalanche photodiodes Low-noise single-photon detection is a prerequisite for quantum information processing using photonic qubits. In particular, detectors that are able to accurately resolve the number of photons in an incident light pulse will find application in functions such as quantum teleportation and linear optics quantum computing. More generally, such a detector will allow the advantages of quantum light detection to be extended to stronger optical signals, permitting optical measurements limited only by fluctuations in the photon number of the source. Here we demonstrate a practical high-speed device, which allows the signals arising from multiple photon-induced avalanches to be precisely discriminated. We use a type of silicon avalanche photodiode in which the lateral electric field profile is strongly modulated in order to realize a spatially multiplexed detector. Clearly discerned multiphoton signals are obtained by applying sub-nanosecond voltage gates in order to restrict the detector current. Many schemes in quantum information processing [1] , [2] , [3] require that the photon number of a detected optical pulse is determined without error. For example, in quantum teleportation [4] and entanglement swapping [5] schemes used in quantum repeaters, a Bell state measurement applied upon two single photons arriving concurrently at a beam splitter requires number states N =0, 1 or 2 to be distinguished in each detector. Similarly, in linear optics quantum computing, the successful operation of a quantum logic gate is often heralded by the detection of a photon number state [6] . Low-noise photon number detection would also be useful for characterizing non-classical light sources [7] , [8] and security analysis in quantum cryptography [9] . In combination with parametric down-conversion sources, photon number detection can also be used for the generation and conditioning of photonic Fock states [10] , as well as more complex quantum light states [11] . Furthermore, many applications beyond pure quantum information processing, such as quantum imaging [12] , tomography [13] , [14] and interferometry [15] , have been suggested to require error-free photon number detection, and extensive efforts [16] , [17] , [18] , [19] , [20] , [21] , [22] , [23] , [24] , [25] , [26] , [27] , [28] , [29] have therefore been devoted to developing photon number resolving detectors. Currently, most of the approaches to photon number detection [16] , [17] , [18] , [19] , [20] require cryogenic cooling, and thus do not address the need for a practical and scalable number resolving detector. In contrast, avalanche photodiodes (APDs) are a mature technology for single-photon detection, which operate close to room temperature, can be fabricated using standard semiconductor processing techniques and are ideal for integration into solid state quantum information processors. As a binary device, APDs used in the so-called Geiger mode, which are also known as single-photon avalanche diodes [21] , have naturally been used as basic building blocks through multiplexing, temporally [22] , [23] , [24] or spatially [25] , [26] , [27] . In particular, silicon photomultipliers are based on high-density arrays of discrete single-photon avalanche diodes, each with their own quenching circuit, which are monolithically integrated into a single chip and coupled electrically using external metallic connections. However, photon number detection realized through multiplexing is not ideal for high-speed operation because of the significant extension in detection time [22] , [23] , [24] or the large RC constants [25] , [26] , [27] . Moreover, significant uncertainty in determining the incident photon number arises from crosstalk effects, long dead times and dark counts. Recently, high-speed photon number detection has been realized using single small-area devices by restricting the avalanche duration [28] , [29] , although statistical noise in the detector output leads to significant uncertainty in the photon number resolution. Here we demonstrate a fast, practical photon number detection using electric field modulation, engineered in a silicon avalanche photodiode (Si-APD). With such modulation, a small-area APD (50×50 μm 2 ) is divided electrically into a few smaller zones that are active for single-photon detection and intrinsically electrically coupled, while retaining the low-device RC constant required for fast gating. Under fast gating, each photon-induced avalanche is allowed to saturate the active zone in which it was stimulated, but the total saturation of the whole device is prevented. Therefore, the output of an electric field-modulated Si-APD consists of contributions from avalanches initiated by photons absorbed in multiple high-field active zones, and indicates the detected photon number. Device structure and microscopy A typical APD comprises a reverse-biased p–n-doped junction, across which a large uniform electric field is generated. In the Geiger mode, for which the breakdown electric field is exceeded, a single photocarrier can trigger a macroscopic current through avalanche multiplication, thus achieving single-photon sensitivity. Conventionally, each avalanche is allowed to grow to a level that saturates the whole device and therefore the detector output does not reflect the number of incident photons. The devices used here are similar to a conventional shallow-junction Si-APD structure [30] , compatible with CMOS (complimentary metal-oxide-semiconductor) processing techniques. 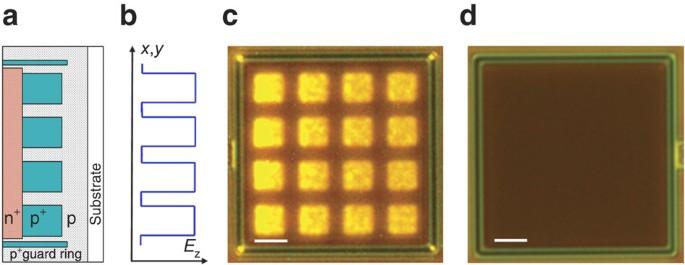Figure 1: Device structure and microscopy. (a) Schematic representation of the lateral doping profile of an electric field-modulated Si-APD, shown in cross-section through the x–y plane. (b) Schematic representation of the lateral electric field profile in the x–y plane. (c) Dark-field emission micrograph, measured for a large dc bias applied beyond the reverse breakdown voltage. The scale bar corresponds to 10 μm. (d) Optical micrograph showing the uniform detector surface, as defined lithographically. The scale bar corresponds to 10 μm. However, a modulated electric field is engineered laterally through the spatial doping distribution in the active plane, as shown schematically in Figure 1a (ref. 31 ). Instead of having a uniform p + -type layer, discrete pockets of highly p + -doped material are separated in the lateral plane by regions of lesser-doped p-type material, formed by successive ion implantations. As a result, the single uniform layer of highly doped n + material used to form the light-sensitive region gives rise to a number of discrete n + –p + junctions within a single small-area diode, that are electrically coupled in parallel through this layer. This modulated doping profile gives rise to the lateral electric field profile shown schematically in Figure 1b . We note that this device structure was originally proposed for reducing the dark count rates in larger area Si-APDs. Figure 1: Device structure and microscopy. ( a ) Schematic representation of the lateral doping profile of an electric field-modulated Si-APD, shown in cross-section through the x–y plane. ( b ) Schematic representation of the lateral electric field profile in the x–y plane. ( c ) Dark-field emission micrograph, measured for a large dc bias applied beyond the reverse breakdown voltage. The scale bar corresponds to 10 μm. ( d ) Optical micrograph showing the uniform detector surface, as defined lithographically. The scale bar corresponds to 10 μm. Full size image Emission microscopy imaging ( Fig. 1c , see Methods for further explanation) reveals the two-dimensional distribution of luminescence to be strongly non-uniform. This is in contrast to the optical micrograph of the detector ( Fig. 1d ), which illustrates that the device consists of a single etched mesa. Regions of bright emission indicate the high-field zones where the electric field across the junction is sufficient to support avalanche multiplication. In photon emission mode, the intermediate low electric field areas between the high-field zones do not contribute strongly to the micrograph as only a linear photocurrent is stimulated. A 4×4 array of high-field zones that are single-photon-sensitive, each being ~9×9 μm 2 , gives a geometrical fill factor for this device of ~50% of the 50×50 μm 2 device area. Single- and multiphoton detection Like an ordinary APD, an electric field-modulated Si-APD would not offer photon number detection when biased conventionally, such that the detector output is allowed to saturate. Therefore, to achieve photon number detection, it is necessary to restrict each avalanche within the high-field zone where it was initiated, and prevent the whole device current from saturating. Under this condition, the raw output of an electric field-modulated APD corresponds to the sum of avalanches initiated by photons absorbed in separate high-field zones, thereby reflecting the photon number in an incident pulse. 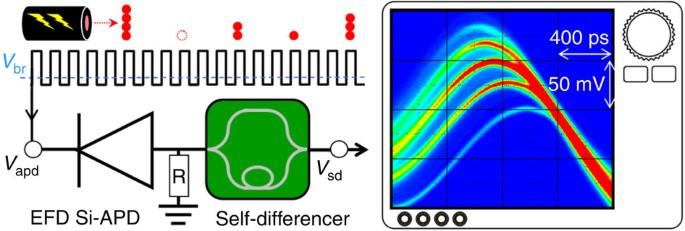Figure 2: Schematic representation of the fast-gated experimental set-up. A bias signal,Vapd, composed of a dc component and a 500-MHz alternating signal is applied to the electric field-modulated Si-APD to periodically bias it above the breakdown voltage,Vbr, and a synchronized laser emits 15-ps pulses at 600 nm. The detector response is sensed as a voltage across a resistor,R, and a self-differencing circuit is used to remove the large capacitive response to the alternating bias signal. The typical output as acquired by a fast oscilloscope is also shown. Here, avalanche restriction is realized using a fast-gated mode, as shown in Figure 2 . A 500-MHz square wave is applied to periodically stimulate the high-field zones into a single-photon-sensitive state. These sub-nanosecond voltage gates are synchronized with 15-ps light pulses at 600 nm, and the device is coupled optically using a 50 μm diameter fibre and a focussing optic to uniformly illuminate the device. The signals are resolved from the capacitive response of the device using a self-differencing circuit [32] (see Methods ). Figure 2: Schematic representation of the fast-gated experimental set-up. A bias signal, V apd , composed of a dc component and a 500-MHz alternating signal is applied to the electric field-modulated Si-APD to periodically bias it above the breakdown voltage, V br , and a synchronized laser emits 15-ps pulses at 600 nm. The detector response is sensed as a voltage across a resistor, R , and a self-differencing circuit is used to remove the large capacitive response to the alternating bias signal. The typical output as acquired by a fast oscilloscope is also shown. Full size image The typical time-resolved voltage output of our detector as measured on an oscilloscope is also shown in Figure 2 , and the output signals of distinctly different amplitude are observed to rise out of the residual capacitive background. We attribute this response to the signals stimulated by quasi-saturated avalanches stimulated in one or more high-field zones, which are summed by the detector due to the electrical coupling through the n + layer, and therefore indicate the number of detected photons. The different detector outputs confirm that the voltage gates are sufficiently short to prevent the total device current from saturating. The progressive displacement in time of the peaks with increasing amplitude is ascribed to the space–charge effect [33] , which reduces the electric field across the junction for each additionally stimulated high-field zone. This arises from the compensation of the ionized donors in the n + layer, owing to the high density of charges in each avalanche. To further investigate the photon number dependence of the electric field-modulated Si-APD, we used an oscilloscope to record the distribution of output voltage pulses obtained from around 5×10 6 samples. 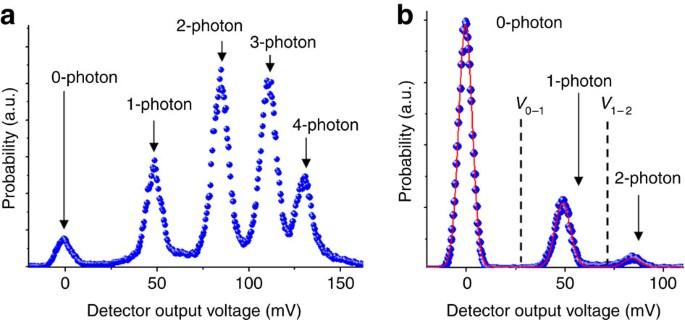Figure 3: Distribution of detector output voltages. (a) Distribution of the output voltage pulses from an electric field-modulated Si-APD, measured for a detected photon fluxμ′=4.8 photons per pulse. (b) Output voltage distribution (symbols) measured for a detected photon fluxμ′=0.92 photons per pulse, for which there are only contributions from 0, 1 and 2 detected photons. The dashed lines correspond to discrimination levels used to determine the photon number error between adjacent photon number states, which are modelled using Gaussian fits (red curves). Figure 3a,b shows the measured probability distribution for detected photon fluxes of μ ′=4.8 and 0.9, respectively (detected per pulse). The peak at 0 mV arises owing to gates in which no photons are detected and the width of this feature corresponds to the electrical noise in the system. The peak at 48 mV is due to the signal stimulated by the detection of a single photon ( N =1) and that at 84 mV is due to two detected photons ( N =2). For the higher flux in Figure 3a , the peaks at 110 and 130 mV arise from N =3 and 4, respectively. The sub-linear dependence of the signal amplitude on N is attributed to the space–charge effect, because of which each additional avalanche will contribute less charge to the total detector current. This effect is also responsible for the absence of any strong features arising from the detection of N ≥5 photons, as the progressive reduction in the electric field prevents avalanche development for high N . Figure 3: Distribution of detector output voltages. ( a ) Distribution of the output voltage pulses from an electric field-modulated Si-APD, measured for a detected photon flux μ ′=4.8 photons per pulse. ( b ) Output voltage distribution (symbols) measured for a detected photon flux μ ′=0.92 photons per pulse, for which there are only contributions from 0, 1 and 2 detected photons. The dashed lines correspond to discrimination levels used to determine the photon number error between adjacent photon number states, which are modelled using Gaussian fits (red curves). Full size image Analysis of photon number statistics The assignment of the output signals to the number of detected photons is further evidenced by the illumination flux dependence. 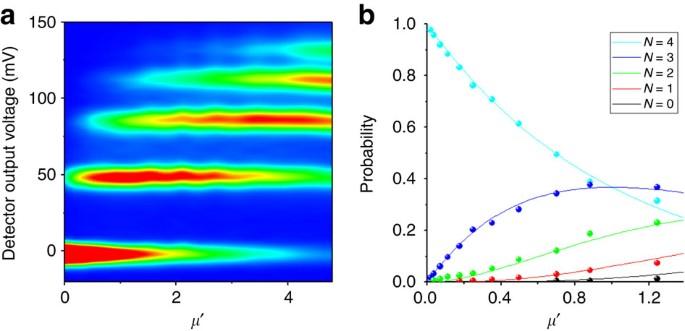Figure 4: Dependence of the detector output on the photon flux. (a) Detected flux dependence of the distribution of output voltage pulses from an electric field-modulated Si-APD. Red corresponds to high intensity and blue to low intensity. (b) Measured occurrence probabilities of theN=0–4 photon peaks (symbols), plotted as a function ofμ′, and the fit obtained using a Poissonian distribution to describe the statistics of the source (lines) for a photon detection efficiency ofη=7.4%. Figure 4a shows the evolution of the detected signal distribution, measured as a function of the detected photon flux, μ ′. As expected, there is only a contribution from the background 'noise' peak in the absence of illumination. For μ ′<0.2 we observe only a single additional peak due to the detection of single photons, which increases in importance as μ ′ is increased further. If we continue to raise the photon flux, the 0- and 1-photon features weaken and a succession of distinct higher voltage peaks emerge and dominate due to the detection of 2, 3 and 4 photons. These features are almost fully discerned and we are therefore able to determine the number of single-photon-induced avalanches very accurately. Figure 4: Dependence of the detector output on the photon flux. ( a ) Detected flux dependence of the distribution of output voltage pulses from an electric field-modulated Si-APD. Red corresponds to high intensity and blue to low intensity. ( b ) Measured occurrence probabilities of the N =0–4 photon peaks (symbols), plotted as a function of μ ′, and the fit obtained using a Poissonian distribution to describe the statistics of the source (lines) for a photon detection efficiency of η =7.4%. Full size image Figure 4b shows the dependence of the occurrence probabilities (symbols) of the N =0, 1, 2, 3 and 4 peaks on μ ′, obtained by fitting the measured voltage distributions with Gaussians. For low-detected photon fluxes, μ ′≤1.4, the occurrence probabilities are very well fitted by Poissonian statistics (solid lines), adjusted to reflect the non-unity detection efficiency of our device, indicating that the measured photon number distribution precisely matches that of the illumination source. For higher detected fluxes the experimental points diverge from the numerical Poissonians, which we attribute to space–charge effects, as described earlier. To establish the photon number detection capability of our device for the measurements used in Bell state analysis, we quantitatively examine the discrimination error in resolving the photon number. Figure 3b shows the output pulse distribution (symbols) obtained for a moderate detected flux μ ′=0.92, giving rise to significant occurrence probabilities for only 0, 1 and 2 photons. The error in determining the detected photon number from the measured output voltage signal, ɛ N , was calculated from the numerical overlap between the Gaussian photon number states (red curves), normalized to reflect a uniform number distribution. We therefore placed single discrimination levels between successive photon numbers for which we obtain discrimination errors ɛ 0 =2.2×10 −10 , ɛ 1 =1.1×10 −4 and ɛ 2 =4.3×10 −5 . Absolute fidelity of photon number detection depends on both the discrimination error and detection efficiency. Electric field-modulated Si-APDs have been shown to discriminate clearly between signals arising from different numbers of single-photon-induced avalanches. This is attributed to the quasi-saturated signals generated within each high-field zone, which negate the statistical effects that increase exponentially with N in conventional fast-gated APDs [28] , [29] . Furthermore, with sub-nanosecond gates, crosstalk between adjacent high-field zones is effectively inhibited, which also improves the fidelity. However, the detection efficiency remains to be improved. Currently, the detection efficiency of the device is measured to be η =7.4%, obtained from the low-flux fit of the measured occurrence probabilities ( Fig. 4b ). Far from unity, this efficiency is a significant source for error in determining the photon number in an incident optical pulse. We note that the single-photon detection efficiency of 7.4% is very low compared with the measured quantum efficiency of 79%, obtained from dc photocurrent measurements. The low single-photon detection efficiency is due to the geometrical fill-factor and, more importantly, a low avalanche initiation probability. The probability for a photocarrier to initiate a macroscopic avalanche depends on both electrical field and thickness of the APD multiplication region. Therefore, improvement in the single-photon detection efficiency can be achieved by device engineering to have higher electric field across a thicker multiplication region. For example, for uniform devices with higher breakdown voltages, the detection efficiency has been demonstrated to approach the quantum efficiency [29] . We expect that the structure of this different type of device could be designed such that the avalanche probability in the high-field regions matches that of uniform devices. In conclusion, we have demonstrated a high-speed photon number detector, realized by a Si-APD with a strongly modulated lateral electric field profile. By applying sub-nanosecond gates to prevent the output signal from saturating, we are able to discriminate signals arising from multiple stimulated high-field zones with high accuracy. We expect the principle of modulating the lateral electric field to be feasible for devices with higher avalanche initiation probabilities, in which case these devices are an excellent prospect for single-shot photon number detection. Owing to the short output signal and the fact that all high-field zones are collectively returned to their initial state during every detector bias cycle, the electric field-modulated Si-APD is particularly suitable for high-speed photon number detection, required for numerous applications in quantum information processing. Emission microscopy In Geiger mode APDs, the large concentration of avalanche carriers in regions of high electric field results in the recombination of a small number of carriers, which are not swept apart by the internal field of the diode. This recombination can occur radiatively, giving rise to breakdown flash [34] and the corresponding luminescent emission in these regions can be clearly observed. The micrographs showing the spatial dependence of the photon emission were measured at room temperature, for which a breakdown voltage V br =28 V was obtained from the reverse current–voltage characteristic. The applied dc voltage of V dc =36 V corresponds to an overbias of 8 V for which a current of 5 mA was generated even in the absence of illumination, therefore indicating the strongly nonlinear gain mode of the detector for these measurements. We used a Nikon Optiphot optical microscope with a ×20 magnification objective, and a high-resolution CCD camera recorded the data in. Fast-gated experiment We applied a detector bias signal consisting of a static dc voltage, V dc , and a 500-MHz alternating component, V ac , to periodically induce an excess voltage above V br , thus stimulating the high-field zones into a single-photon-sensitive state. For these experiments the sample was cooled thermo-electrically to −30 °C, for which the breakdown voltage was V br =27 V. The applied dc voltage V dc =29.4 V is therefore greater than V br , requiring a square wave gate of amplitude of V ac ~6 V to quench the avalanche photocurrent during the low bias part of the detector bias cycle. Photon-induced avalanches generate a current through the APD that is sensed as a voltage across the 50 Ω resistor. The rapidly alternating bias induces a strong background signal across the resistor due to the rapid charging and discharging of the APD. In order to detect the weak unsaturated signal arising from sub-nanosecond voltage gates, we remove this capacitive component using a self-differencing circuit. This subtracts the gated APD output from that in the preceding period, leaving only the avalanche response of the detector and a comparatively weak residual signal due to any uncancelled component of the capacitive response. We minimize this component by accurately tuning the delay between the two signals and also impedance-matching the signal arms. Measurement of detected photon flux The optical excitation for the following experiments was obtained using sum frequency generation between 1,550-nm laser pulses of 15-ps duration and a 980-nm continuous-wave pump laser. The up-converted 600-nm photons were synchronized at 1/32 of the gate frequency (500 MHz/32), and the signal was attenuated to the incident photon flux, μ , measured per pulse using a calibrated optical power metre. The detected flux was subsequently calculated using the single-photon detection efficiency, η =7.4%, determined from the flux dependence of the measured occurrence probabilities. This value was verified by the single-photon detection probability obtained from the detector voltage distribution for an incident flux, μ =0.1, for which only 0- and 1-photon events contribute. How to cite this article: Thomas, O. et al . Practical photon number detection with electric field-modulated silicon avalanche photodiodes. Nat. Commun. 3:644 doi: 10.1038/ncomms1641 (2012).